Association analysis identifies new risk loci for congenital heart disease in Chinese populations Our previous genome-wide association study (GWAS) identified two susceptibility loci for congenital heart disease (CHD) in Han Chinese. Here we identify additional loci by testing promising associations in an extended 3-stage validation consisting of 6,053 CHD cases and 7,410 controls. We find GW significant ( P <5.0 × 10 −8 ) evidence of 4 additional CHD susceptibility loci at 4q31.22 (rs1400558, upstream of EDNRA , P all =1.63 × 10 −9 ), 9p24.2 (rs7863990, close to SMARCA2 , P all =3.71 × 10 −14 ), 12q24.13 (rs2433752, upstream of TBX3 and TBX5 , P all =1.04 × 10 −10 ) and 20q12 (rs490514, in PTPRT , P all =1.20 × 10 −13 ). Moreover, the data from previous European GWAS supports that rs490514 is associated with the risk of CHD ( P =3.40 × 10 −3 ). These results enhance our understanding of CHD susceptibility. Congenital heart disease (CHD) is currently the most common birth defect worldwide. Twenty-eight per cent of all major congenital anomalies consist of heart defects [1] . Epidemiologically, the worldwide prevalence of CHD is estimated to be 8 per 1,000 live births [1] , [2] , [3] and 4 per 1,000 adults [4] . CHD is also a leading cause of perinatal and infant mortality, causing more than 220,000 deaths globally every year [5] . In addition, patients with CHD often need long-term and high-cost medical care [6] . CHD may occur as a part of many recognized chromosomal and Mendelian syndromes [7] , [8] , however, in 75% of cases it manifests as a non-syndromic condition and may result from a multifactorial inheritance model that involves a multitude of susceptibility genes with low- (common variants) or intermediate-penetrance mutations (rare variants) [9] . To date, several genome-wide association studies (GWASs) have achieved success in deciphering the genetic basis of CHD [10] , [11] , [12] . One study on European Caucasians reported that single nucleotide polymorphisms (SNPs) at chromosome 4p16 were associated with the risk of atrial septal defect (ASD), but not other subtypes [11] . Simultaneously, we reported a multistage GWAS of CHD in Han Chinese and identified two CHD susceptibility loci (rs2474937 at 1p12 for TBX15 and rs1531070 at 4q31.1 for MAML3 ) [10] . Additional genetic factors, particularly those with relatively moderate P values in the GWA scan, still remain to be discovered. Here we conduct an evaluation of the promising associations in an extended 3-stage replication, using 6,053 unrelated CHD cases and 7,410 non-CHD controls, and focus on the SNPs that had P values ranging from 10 −4 to 10 −5 in the GWA scan ( Supplementary Fig. 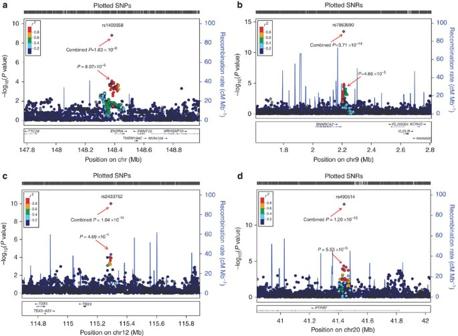Figure 1: Regional plot of the four identified lead SNPs. These SNPs are (a) rs1400558 at 4q31.22, (b) rs7863990 at 9p24.2, (c) rs2433752 at 12q24.13 and (d) rs490514 at 20q12. The results (−log10P) are shown for the SNPs located in the 600-kb region flanking either side of the marker SNPs in the GWA scan stage. Genetic association testing was performed using logistic regression analyses under an additive model. First principal component was adjusted in GWA scan stage. The marker SNPs are shown as purple circles with theirPvalues in GWA scan stage and as purple diamonds with theirPvalues in the combined stage when all of the CHD cases and non-CHD controls from the GWA scan and Validations I, II and III were pooled together. Ther2values of the remaining SNPs are indicated by different colours. The genes within the region-of-interest are annotated, with arrows indicating the direction of transcription. For each plot, the recombination rates (righty-axes) of the region are shown according to their chromosomal positions (x-axis). 1 , Supplementary Table 1 and Supplementary Data 1 ).We find evidence of four new CHD susceptibility loci at 4q31.22 (rs1400558, upstream of endothelin receptor type A ( EDNRA ), P all =1.63 × 10 −9 ), 9p24.2 (rs7863990, close to SWI/SNF-related, matrix-associated, actin-dependent regulator of chromatin, subfamily a, member 2 ( SMARCA2 ), P all =3.71 × 10 −14 ), 12q24.13 (rs2433752, upstream of T-box 3 ( TBX3 ) and T-box 5 ( TBX5 ), P all =1.04 × 10 −10 ) and 20q12 (rs490514, in protein tyrosine phosphatase, receptor type, T ( PTPRT ), P all =1.20 × 10 −13 ). Using data from previous European GWAS, we find that rs490514 is also associated with the risk of CHD ( P =3.40 × 10 −3 ), but no significant association was observed for rs1400558. Susceptibility loci of CHD in validation studies For the GWAS scan stage, we analysed association between CHD and 708,275 SNPs in 945 CHD cases and 1,246 control individuals in an additive model using logistic regression analyses with adjustment for the top eigenvector. Forty-five SNPs met the selection criteria for the first-stage validation (Validation I) ( Table 1 and Supplementary Data 1 ). We performed logistic regression analysis under an additive model of the validation samples. In Validation I, 4 SNPs at 4q31.22 (rs1400558), 9p24.2 (rs7863990), 12q24.13 (rs2433752) and 20q12 (rs490514) were consistently replicated in 2,770 ASD, ventricular septal defect (VSD) and ASD combined VSD (the occurrence of an ASD together with a VSD) cases and 3,911 controls from Nanjing. For the second-stage validation (Validation II), additional 1,095 cases with ASD, VSD or ASD combined VSD and 2,379 controls from Xi’an were genotyped to verify the significant associations of the 4 loci, and they were all consistently associated with CHD risk ( Table 1 and Supplementary Data 1 ). Moreover, the associations of the 4 SNPs were evaluated in 1,437 CHD cases from Nanjing and 751 CHD cases from Xi’an that had phenotypes different from those of isolated ASD, isolated VSD or ASD combined VSD, using 773 controls from Nanjing and 347 controls from Xi’an referred to as Validation IIIa and Validation IIIb, respectively. A meta-analysis of Validation IIIa and Validation IIIb was conducted to evaluate the association in a total of 2,188 CHD cases with phenotypes that were different from isolated ASD, isolated VSD or ASD combined VSD, and in 1,120 controls, and the significant associations were still observed (odds ratio (OR)=1.18, P =2.91 × 10 −3 for rs1400558; OR=1.45, P =1.76 × 10 −5 for rs7863990; OR=0.82, P =1.23 × 10 −3 for rs2433752; and OR=1.22, P =1.96 × 10 −4 for rs490514) ( Table 1 and Supplementary Data 1 ). Table 1 Associations of 4 SNPs to CHD in the GWA scan and validation studies. Full size table Combined analysis of the susceptibility loci In the combined analysis, additive model of logistic regression analyses were used to estimate the P values of association analyses. We first pooled all of the ASD, VSD and ASD combined VSD cases and non-CHD controls. All 4 SNPs reached GW significance ( P <5.0 × 10 −8 ) for CHD susceptibility (OR=1.17, P all =2.75 × 10 −9 for rs1400558; OR=1.29, P all =7.47 × 10 −9 for rs7863990; OR=0.80, P all =1.80 × 10 −11 for rs2433752; and OR=1.19, P all =3.53 × 10 −11 for rs490514) ( Table 1 ). In addition, all of the CHD cases and non-CHD controls from the GWA scan and Validations I, II and III were pooled together. Once again, all four SNPs demonstrated significant GW associations (OR=1.15, P all =1.63 × 10 −9 for rs1400558; OR=1.34, P all =3.71 × 10 −14 for rs7863990; OR=0.83, P all =1.04 × 10 −10 for rs2433752; and OR=1.19, P all =1.20 × 10 −13 for rs490514) without significant heterogeneity between the stages ( Table 1 ). Stratified analysis by diagnostic groups In a stratified analysis, we evaluated the associations of the four SNPs using logistic regression analysis under additive model in the major subtypes of ASD, VSD, ASD combined VSD, patent ductus arteriosus (PDA) and tetralogy of fallot (TOF). The heterogeneity between subgroups was assessed with the χ 2 -based Cochran’s Q test. Heterogeneities in the ORs for rs1400558 and rs7863990 were observed among the different subtypes ( P =0.015 and 0.007, respectively) ( Table 2 ). For the other two SNPs (rs2433752 and rs490514), the association strengths were not significantly different among the five subtypes ( P =0.249 and 0.193, respectively) ( Table 2 ). Rs1400558 showed significant associations with all subtypes except PDA (OR=0.88, P =1.24 × 10 −1 ). The SNP rs7863990 exhibited significant associations in all of the CHD subtypes, and the strongest association was with the TOF subtype (OR=1.76, P =5.39 × 10 −7 ). For rs2433752, although no significant association was observed in PDA subgroup, similar effect sizes were observed for all subtypes including PDA. For rs490514, significant associations were only seen in ASD, VSD and ASD combined VSD groups. Table 2 Stratified analysis by major subtypes of CHD for the 4 identified SNPs. Full size table Association analysis in European CHD GWAS Cordell et al . [11] published two studies of CHD in Europeans, one of them recruited multiple CHD phenotypes and the other one only included TOF cases [12] . Using their existing GWA scan data, we attempted to investigate the associations of the four SNPs we identified and the CHD risk in Europeans. We pooled all samples of these two studies together and evaluated the associations using logistic regression analysis under additive model. Two SNPs (rs1400558 and rs490514) were genotyped in their data. We found that rs490514 is associated with the risk of CHD significantly in Europeans (OR=1.18, P =3.40 × 10 −3 ), while no significant association was observed for rs1400558 (OR=1.02, P =6.18 × 10 −1 ) ( Table 3 ). We also carried out subsidiary analyses for these two SNPs in six different diagnostic groups: ASD, VSD, transposition of the great arteries (TGA), conotruncal malformations, left-sided malformations and TOF. The association strengths were not significantly different among different subtypes ( P =0.700 and 0.908, respectively) ( Supplementary Table 2 ). Table 3 Associations of 2 SNPs to CHD in European GWAS data. Full size table Imputation analysis An imputation analysis in our GWA scan samples identified the associations of the SNPs with CHD risk at P ≤1.0 × 10 −4 (imputed r 2 >0.3, quality threshold>0.9, minor allele frequency (MAF)>0.05, located 500 kb up- or downstream of the four lead SNPs). For 4q31.22, we did not identify any untyped SNPs in high linkage disequilibrium (LD) with the lead SNP that reached P ≤1.0 × 10 −4 ( Fig. 1a and Supplementary Table 3 ). For 9p24.2, a series of SNPs reaching P ≤1.0 × 10 −4 were in strong LD with rs7863990 (four SNPs: r 2 =0.81-0.90, P =1.46 × 10 −5 to 2.86 × 10 −5 , Fig. 1b and Supplementary Table 3 ). Rs2433748 was in high LD with rs2433752 at 12q24.13 ( r 2 =0.86, P =9.92 × 10 −5 , Fig. 1c and Supplementary Table 3 ). In addition, we found 2 SNPs in high LD with rs490514 at 20q12 ( r 2 =1.00 for rs13039258, P =5.33 × 10 −5 and r 2 =0.95 for rs6103054, P =6.84 × 10 −5 , Fig. 1d and Supplementary Table 3 ). Figure 1: Regional plot of the four identified lead SNPs. These SNPs are ( a ) rs1400558 at 4q31.22, ( b ) rs7863990 at 9p24.2, ( c ) rs2433752 at 12q24.13 and ( d ) rs490514 at 20q12. The results (−log 10 P ) are shown for the SNPs located in the 600-kb region flanking either side of the marker SNPs in the GWA scan stage. Genetic association testing was performed using logistic regression analyses under an additive model. First principal component was adjusted in GWA scan stage. The marker SNPs are shown as purple circles with their P values in GWA scan stage and as purple diamonds with their P values in the combined stage when all of the CHD cases and non-CHD controls from the GWA scan and Validations I, II and III were pooled together. The r 2 values of the remaining SNPs are indicated by different colours. The genes within the region-of-interest are annotated, with arrows indicating the direction of transcription. For each plot, the recombination rates (right y -axes) of the region are shown according to their chromosomal positions ( x -axis). Full size image Our three-stage validation provides compelling evidence that four new SNPs at 4q31.22 (rs1400558, upstream of EDNRA ), 9p24.2 (rs7863990, close to SMARCA2 ), 12q24.13 (rs2433752, upstream of TBX3 and TBX5 ) and 20q12 (rs490514, within the second intron of PTPRT ) influence the risk of CHD in Chinese populations. EDNRA , SMARCA2 , TBX3 and TBX5 have been implicated to be involved in heart development in multiple previous studies. Moreover, the data of previous European GWAS supports that rs490514 is also associated with the risk of CHD in Europeans. On chromosome 20, rs490514 is located within the second intron of protein-tyrosine phosphatase receptor type T ( PTPRT ). PTPRT is a member of the PTP family [13] . PTPs are known to be signalling molecules that regulate a variety of cellular processes, including cell growth, differentiation, the mitotic cycle and oncogenic transformation. Their protein domain structures suggest their roles in both signal transduction and cellular adhesion [14] , [15] . Many members of the PTP family are expressed in various tissues, including the heart [15] . Although Zhao et al . [16] , found no obvious developmental abnormalities in homozygous PTPRT knockout mice, it is possible that it functions in certain genetic background or environmental conditions [17] . Combinations of a heterozygous missense mutation at the conserved PTP catalytic domain of PTPRT and a heterozygous intronic deletion of 150 kb removing more than half of intron 1 of PTPRT were reported in a Dutch family of three brothers and two sisters affected with intellectual disability, together with congenital cardiac defects [18] , indicating possible essential function of PTPRT in heart development. In addition, using European GW scan data, we found that rs490514 is also associated with the risk of CHD in Europeans, although the allele frequency of rs490514 in both populations was greatly different (Chinese population: MAF=0.39 in controls; European population: MAF=0.11 in controls). The SNP rs2433752 is located 170 kb and 448 kb upstream of T-box 3 ( TBX3 ) and T-box 5 ( TBX5 ), respectively. The T-box genes encode important transcription factors involved in the regulation of developmental processes, such as heart development. These genes often act in a combinatorial manner and exhibit an exquisite dose sensitivity when controlling heart developmental processes [19] , [20] . In the human heart, TBX3 is expressed in the atrial floor and atrioventricular canal myocardium [21] . Various cardiac defects, such as VSD, double outlet right ventricle and TGA, have been observed in Tbx3-deficient model animals [22] , [23] , [24] . Another nearby gene, TBX5 , plays important roles in chamber formation, septation and cardiomyocyte differentiation [25] . Both gain- and loss-of-function experiments on Tbx5 have resulted in abnormal heart phenotypes in animal models, such as looping defects, loss of the ventricular septum and arrested development of the AV cushions, hypoplastic sinoatrial region and left ventricle [26] , [27] . The polymorphisms in the upstream region potentially influence the transcriptional activity, and the haplo-insufficiency of TBX3 and TBX5 has also been proven to be associated with CHD [28] , [29] . The SNP rs7863990 localizes 17 kb downstream of SMARCA2 . The encoded protein of SMARCA2 is part of the Brg1/Brm-associated factor (BAF) chromatin remodelling complex, which is thought to regulate the transcription of certain genes by altering chromatin structure [30] . Each BAF complex utilizes either SMARCA4 (also known as BRG1) or SMARCA2 (also known as BRM) as alternative catalytic subunits [31] . TBX5, Nkx2-5 and GATA4 interact with BAF complexes, and this interaction is important for the de novo induction of cardiac differentiation from embryonic mesoderm [32] , [33] . The disruption of the delicate balance between certain transcription factors and the BAF complexes is likely to be a mechanistic cause of CHD [34] . Some studies have revealed that Smarca4 is essential for heart development in mouse and zebrafish embryogenesis, whereas Smarca2 appears to be dispensable [34] , [35] . In humans, the role of SMARCA2 in cardiogenesis is unclear; however, several independent exome sequencing projects have identified de novo mutations in SMARCA2 that are associated with two congenital syndromes that include cardiac defects: Coffin–Siris syndrome and Nicolaides–Baraitser syndrome [36] , [37] . We also identified associations between rs1400558 and CHD among Chinese. This SNP is located 22 kb upstream of endothelin receptor type A ( EDNRA ). In expression quantitative trait locus (eQTL) analysis using GTEx Portal ( http://www.gtexportal.org/home/ ), we found the risk allele (A) of rs1400558 was significantly associated was lower mRNA expression of EDNRA in 86 heart left ventricle tissues ( P =0.0079), while no eQTL effects were identified for the other 3 SNPs. In the mouse model, a subpopulation of the first (crescent forming) heart field has been shown to be marked with Ednra gene expression [38] . Furthermore, Ednra-mediated signals are involved in myocardial growth, ventricular formation and aortic arch patterning [38] , [39] . It has been reported that the mice deficient in Ednra signalling exhibit aortic arch malformation and outflow anomalies [39] , [40] . In addition, Ednra -null embryonic hearts often demonstrate hypoplasia of the ventricular wall, low mitotic activity and decreased Tbx5 expression with reciprocal expansion of Tbx2 expression [38] . However, in European GWA scan data, no significant association was observed for rs1400558 and the risk of CHD and the allele frequency of this SNP in Chinese and Europeans also showed difference. There might be different lead SNP for Europeans in this region because of underlying genetic heterogeneity, which merits further investigations. In a stratified analysis, heterogeneity of the association strengths was observed among the different subtypes of CHD. For the SNP rs1400558, similar associations were observed in the ASD, VSD, ASD combined VSD and TOF subtypes but not in PDA, which could be due to the susceptibility gene EDNRA , which was reported to be involved in the formation of the ventricles rather than the ductal media. In all of the CHD subtypes, rs7863990 exhibited significant associations, and the strongest association was with the TOF subtype. Studies have reported that BAF complexes interact with many important transcription factors, such as TBX5, Nkx2-5 and GATA4, and may further play essential roles in the formation of the outflow tract. Although no significant association was observed between rs2433752 and PDA, the sample size of this group was relatively small, and the effect size was comparable to VSD. For rs490514, the associations were not different between the subtypes. As the sample size of the PDA and TOF groups was relatively small compared with the other three groups, further studies with larger sample populations are highly recommended. In conclusion, we identified four new CHD susceptibility loci at 4q31.22, 9p24.2, 12q24.13 and 20q12 in Han Chinese, by performing the extended three-stage validation. These findings further advance our understanding of the susceptibility to CHD. Study design This study was approved by the institutional review boards of Nanjing Medical University and The Fourth Military Medical University. All participants completed the informed consent in writing before taking part in this research. We performed a four-stage case-control analysis. The GWAS phase included 945 CHD cases and 1,246 non-CHD controls recruited from the First Affiliated Hospital of Nanjing Medical University and the Affiliated Nanjing Children’s Hospital of Nanjing Medical University (Nanjing, China) between March 2006 and March 2009. For the first-stage validation (Validation I), 2,770 cases and 3,911 controls were recruited from the two hospitals above between March 2006 and June 2013. For the second-stage validation (Validation II), 1,095 cases and 2,379 controls were recruited from Xijing Hospital (Xi’an, China). In addition, 1,437 and 751 CHD cases with phenotypes different from isolated ASD, VSD or ASD combined VSD were recruited from the First Affiliated Hospital of Nanjing Medical University and the Affiliated Nanjing Children’s Hospital of Nanjing Medical University (Validation IIIa) and the Xijing Hospital (Validation IIIb), respectively. The Validation IIIa and IIIb included 773 and 347 non-CHD controls from the hospitals in Nanjing and Xi’an above, respectively. We summarized all subjects in Supplementary Tables 1 and 4 . All of the samples used in the validations in the previous study [10] were included in the current study. Non-syndromic CHD cases were diagnosed on the basis of echocardiography; and some diagnoses were further confirmed by cardiac catheterization and/or surgery (detailed classifications are shown in Supplementary Table 4 ). CHD cases that manifested additional syndromes, multiple developmental abnormalities or known chromosomal abnormalities were excluded from the study. We next excluded cases if they had positive family history of CHD in their first-degree relatives or if their mothers had maternal diabetes mellitus, phenylketonuria, teratogen exposure or therapeutic drug exposure during pregnancy. All of the controls were non-CHD outpatients who were recruited from the hospitals above over the same time period. Subjects exhibiting congenital anomalies or cardiac disease were excluded from the control group. For each participant, ∼ 2 ml of whole blood was obtained to extract genomic DNA for genotyping analysis. The discovery cohorts of the two European GWASs comprise CHD cases of multiple phenotypes and TOF cases [11] , [12] . All cases are self-reported European Caucasian ancestry recruited from multiple centres in the UK and from centres in Leuven, Belgium, Erlangen, Germany and Sydney, Australia. SNP genotyping in the cases was carried out using the Illumina Human660W-Quad array, and genotypes were compared with data for UK population-based controls (genotyped on the Illumina 1.2M chip) obtained from the Wellcome Trust Case Control Consortium 2 (WTCCC2). All diagnoses were established by CHD specialists at the contributing centres, and cases were classified using European Paediatric Cardiac Codes. Cases exhibiting clinical features of recognized malformation syndromes, multiple developmental abnormalities or learning difficulties were excluded from the study [11] , [12] . After stringent quality control, we analysed the associations of two typed SNPs (rs1400558 and rs490514) and the risk of CHD in the current data set which consisted of 2,111 unrelated CHD cases (ASD: 340; VSD: 191; TGA: 207; conotruncal malformations: 151 and left-sided malformations: 387; TOF: 835) and 5,159 controls. SNP selection and genotyping for validation The SNPs for Validation I were selected based on the following criteria: (i) the SNPs had 1.0 × 10 −5 < P ≤1.0 × 10 −4 in the GWAS stage; (ii) the SNPs were not located in the same chromosomal region/gene of SNPs reported in our previous study [10] ; (iii) the SNPs had clear genotyping clusters; (iv) if more than one SNPs were located in the same chromosomal region/gene, only one SNP with the lowest P value was selected; and (v) only the SNP with the lowest P value was selected when multiple SNPs were observed in strong LD ( r 2 ≥0.8). A total of 45 SNPs met these criteria ( Supplementary Data 1 ). Significantly associated SNPs ( P <0.05) were further genotyped in validation samples. Genotyping was performed using the iPLEX Sequenom MassARRAY platform (Sequenom, Inc., USA) in Validation I and the TaqMan Allelic Discrimination Assay (Applied Biosystems, Inc., USA) in Validation II and III. The primers of nine SNPs using TaqMan allelic discrimination Assay to perform genotyping were provided in Supplementary Table 5 The details of primers and probes used for TaqMan allelic discrimination assay in validation stage were provided in Supplementary Table 5 . We controlled the quality of genotyping based on the following methods: (i) case and control samples were mixture distributed on each 384-well plate; (ii) genotyping was carried out using blind method; (iii) positive and negative controls were included in each plate; and (iv) 5% randomly selected samples were repeat genotyping to calculate the coincidence rate. Statistical analysis The association analysis was performed using an additive model in a logistic regression analysis in PLINK 1.07 ( http://pngu.mgh.harvard.edu/~purcell/plink/ ). The heterogeneity between subgroups was assessed with the χ 2 -based Cochran’s Q test. The meta-analysis was performed in a combined analysis, and a random-effects model was used when heterogeneity between the studies existed (if the P value for the heterogeneity test was <0.05), otherwise, a fixed-effect model was used. We used MACH 1.0 software ( http://www.sph.umich.edu/csg/abecasis/MACH/ ) to impute the ungenotyped SNPs using the LD information from the hg18/1000 Genomes Project database (CHB+JPT as a reference set; June 2010 release). The chromosomal region was plotted using LocusZoom 1.1 ( http://csg.sph.umich.edu/locuszoom/ ). All of the other analyses were performed with R software 2.15.1 ( http://www.r-project.org./ ). How to cite this article: Lin, Y. et al . Association analysis identifies new risk loci for congenital heart disease in Chinese populations. Nat. Commun. 6:8082 doi: 10.1038/ncomms9082 (2015).